Visualizing the interfacial evolution from charge compensation to metallic screening across the manganite metal–insulator transition Electronic changes at polar interfaces between transition metal oxides offer the tantalizing possibility to stabilize novel ground states yet can also cause unintended reconstructions in devices. The nature of these interfacial reconstructions should be qualitatively different for metallic and insulating films as the electrostatic boundary conditions and compensation mechanisms are distinct. Here we directly quantify with atomic-resolution the charge distribution for manganite–titanate interfaces traversing the metal–insulator transition. By measuring the concentration and valence of the cations, we find an intrinsic interfacial electronic reconstruction in the insulating films. The total charge observed for the insulating manganite films quantitatively agrees with that needed to cancel the polar catastrophe. As the manganite becomes metallic with increased hole doping, the total charge build-up and its spatial range drop substantially. Direct quantification of the intrinsic charge transfer and spatial width should lay the framework for devices harnessing these unique electronic phases. The interface between transition metal oxides is a playground for stabilizing novel phases not apparent in the parent compounds [1] , [2] , [3] , [4] , [5] , [6] , [7] . This is evidenced by the observation of conductivity [1] and later superconductivity [4] and magnetism [8] at the interface between two non-magnetic insulators LaAlO 3 and SrTiO 3 as well as novel magnetic phases [2] and correlated electron phases [7] . Manganites, such as La 1− x Sr x MnO 3 , exhibit many of the exotic bulk phases seen in the complex oxides, with paramagnetic insulating ( x≤ 0.2) and ferromagnetic metallic ground states ( x> 0.2) at room temperature and additional charge and orbital ordered phases accessible at low temperatures [9] , [10] . Next generation spin tunnel junctions could be formed by exploiting the room temperature ferromagnetism in ultrathin layers of La 0.67 Sr 0.33 MnO 3 (ref. 11 ). Observed interfacial dead layers have, however, limited the scaling of potential devices [12] , [13] , [14] . While explicit attempts [15] , [16] to offset the interface dipole [17] , [18] and to eliminate extrinsic defects [14] have reduced the observed dead layer thickness, direct mapping of these intrinsic electronic and magnetic reconstructions at the interface can be obscured by variations in growth techniques leading to competing defects. The intrinsic reconstructions at the interface between an insulating polar film and non-polar substrate, for example a LaMnO 3 film on a SrTiO 3 {100} substrate, are typically thought of in terms of the polar catastrophe model [19] , [20] : the presence of alternating positively and negatively charged layers on a non-polar surface causes the build-up of a non-zero electric field and an electric potential, which diverges with sample thickness. The polar catastrophe can be alleviated by transferring charge to the interface—manifest as either the presence of an extra half of an electron or hole at an n- type (LaO/TiO 2 ) and p- type (MnO 2 /SrO) interface, respectively—yet also through cation or oxygen vacancies and/or atomic displacements [21] . Note that oxygen vacancies in SrTiO 3 , for example, can give rise to itinerant electrons [22] , [23] yet can only cancel the polar catastrophe for p- type interfaces [20] . For metallic and insulating films, the nature of the interfacial reconstructions should be qualitatively different as the electrostatic boundary conditions and compensation mechanisms are distinct. Some metal/semiconductor oxide interfaces, for example metallic non-polar SrRuO 3 films on SrTiO 3 substrates [24] , can be well described as ideal Schottky barriers. Others, such as conducting polar La 1-x Sr x MnO3/SrTiO 3 interfaces [15] , [24] , require additional dipoles to compensate for the interface charge. This interface dipole could take the form of an extra screening charge or atomic displacements of the constituent atoms. Studying these electronic reconstructions at La 1-x Sr x MnO 3 /SrTiO 3 /SrTiO3 interfaces provides an ideal platform to probe the interface across the manganite metal–insulator transition. The large changes in electronic properties are induced by continuous hole doping while maintaining the same crystal topology via the Mn-O backbone. The interfacial changes in the composition and bonding information can be exquisitely probed at the atomic-scale with scanning transmission electron microscopy (STEM) in combination with electron energy loss spectroscopy (EELS) [25] . In the single-particle picture, the energy loss due to inelastic scattering from core-level transitions provides a site-specific measurement of the local density of states above the Fermi level, partitioned by chemical species and angular momentum due to the dipole selection rules [26] . For transition metal L 2,3 edges of relevance for probing the multivalent titanium and manganese atoms, however, strong core-hole effects produce a significant deviation between the local density of states and the observed energy loss near edge fine structure [26] . Nevertheless, comparison with reference spectra has permitted atomic-resolution two-dimensional mapping of oxidation states [27] , [28] , [29] . Here, we provide a systematic study of a series of La 1− x Sr x MnO 3 /Nb:SrTiO 3 (‘LSMO’/‘STO’) interfaces from x =0 to x =0.5, prepared under identical growth conditions, to disentangle the extrinsic and intrinsic effects at the interface through a range of states on the manganite phase diagram. By measuring the concentration and valence of all cations in the system using EELS, we explicitly quantify the electronic charge transfer apparent as a cation valence change. We show a quantitative agreement between the polar catastrophe model and the total electron transfer to the manganese sites of the insulating LSMO films, yet a considerable drop in the total charge transfer and spatial extent with the onset of screening in the metallic La 0.7 Sr 0.3 MnO 3 . Elemental mapping of the La 0.9 Sr 0.1 MnO 3 /SrTiO 3 interface We investigate thin films of La 1− x Sr x MnO 3 with x =0, 0.1, 0.2, 0.3 and 0.5 grown on SrTiO 3. To demonstrate the ability of EELS to chemically map valence changes, interdiffusion and vacancies at atomic-resolution, we first investigate the La 0.9 Sr 0.1 MnO 3 /SrTiO 3 interface. The high-angle annular dark-field STEM image shown in Fig. 1a indicates that the interface is coherent and free of dislocations. From the EELS elemental maps in Fig. 1b–e , we note an asymmetry in cation intermixing as the ‘ B -site’ manganese/titanium sublattice only shows one monolayer of intermixing, while the ‘ A -site’ lanthanum shows considerable interdiffusion over approximately four monolayers ( Supplementary Fig. 1 ). The polar discontinuity shown in Fig. 1f and Supplementary Fig. 2 cannot be alleviated by A -site interdiffusion in and of itself, however, asymmetric diffusion could reduce (or enhance) the interfacial potential offset ( Supplementary Fig. 3 ). Surprisingly though, preferential diffusion between the A -site cations for the La 0.9 Sr 0.1 O/TiO 2 interface without changes in the B -site cation valence serves to increase the potential build-up rather than decrease it. On the other hand, cation vacancies could provide negatively charged defects to reduce the potential build-up in the film [30] , [31] . Despite the observed asymmetric interdiffusion, the total cation concentration across the interface does not deviate by more than 3±5% from that of a cation ‘vacancy-free’ interface, even for the most diffuse interface, as shown in Supplementary Figs 4 and 5 . There are mechanisms whereby local deviations from stoichiometry can alter the local cation valence. For instance, Mn +2 could substitute on the La (Sr) site in La-deficient LaxMnO3-δ (refs 32 , 33 ). From the measured deviations in (La+Sr) composition profiles, this could account for up to 3±5% of the A -sites, or up to 6±11% of the Mn +2 that we observe spectroscopically. Therefore, extrinsic defect-driven mechanisms, while possibly present, do not play a dominant role in our films. 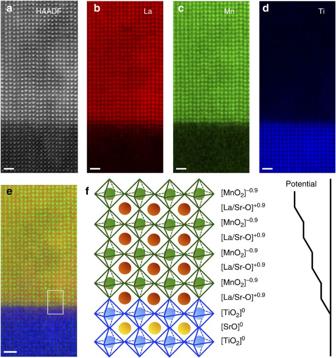Figure 1: EELS spectroscopic mapping of the La0.9Sr0.1MnO3/SrTiO3interface. Simultaneously recorded high-angle annular dark-field STEM image (a) and false-colour La, Mn and Ti elemental concentration maps (b–d) of the interface. (e) Combined elemental map with Ti in blue, Mn in green and La in red. (f) Cartoon of an atomically abrupt La0.9Sr0.1MnO3/SrTiO3interface with the diverging electric potential due to the polar discontinuity at the interface. A corresponding area in the spectroscopic map is indicated by a white box in (e). Scale bar, 1 nm. Figure 1: EELS spectroscopic mapping of the La 0.9 Sr 0.1 MnO 3 /SrTiO 3 interface. Simultaneously recorded high-angle annular dark-field STEM image ( a ) and false-colour La, Mn and Ti elemental concentration maps ( b – d ) of the interface. ( e ) Combined elemental map with Ti in blue, Mn in green and La in red. ( f ) Cartoon of an atomically abrupt La 0.9 Sr 0.1 MnO 3 /SrTiO 3 interface with the diverging electric potential due to the polar discontinuity at the interface. A corresponding area in the spectroscopic map is indicated by a white box in ( e ). Scale bar, 1 nm. Full size image Charge mapping at the La 0.9 Sr 0.1 MnO 3 /SrTiO 3 interface As the polar discontinuity was not alleviated by cation vacancies, we now turn to charge modulation. The Mn-L 2,3 edge binned parallel to the interface is shown in Fig. 2a ; near the interface the major peaks shift to lower energies, indicative of a reduced manganese valence state. From this edge, two distinct components were extracted with multivariate curve resolution—a bulk Mn +3.1 spectra and a lower valence state—as shown in Fig. 2b . A non-negative non-linear least squares fit to the full Mn-L 2,3 edge reveals the presence of a significant fraction of a lower valence state at the interface as shown in the binned line profile in Fig. 2c and full 2-D fit in Fig. 2d . The residual from the fit is presented in Supplementary Figs 6 and 7 . A similar analysis of titanium did not yield a change in the valence below the nominal Ti +4 of bulk SrTiO 3 as discussed in Supplementary Fig. 8 . This indicates that the majority of the electronic transfer to the interface resides on the manganese sites in our samples rather than titanium sites as was claimed for LaMnO 3 /SrTiO 3 superlattices [34] . Note that diffusion of a manganese atom onto a titanium site should drive the manganese valence up from the nominal bulk valence of +3.1 towards the titanium valence of +4. Experimentally, however, we show that the interfacial manganese valence instead decreases. Similarly, intermixing on the A -site, as observed in Supplementary Fig. 5 , would place Sr atoms on the La sites in the LSMO films. Without changes in the B -site cation valence, this once again would serve to increase the interfacial manganese valence, in contrast to the experimentally observed decrease. Thus, the changes in manganese valence observed cannot be interpreted by interdiffusion-driven valence changes. 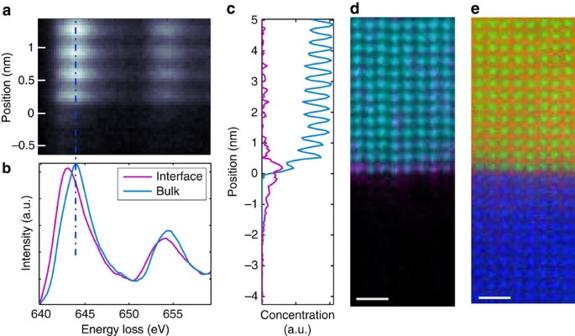Figure 2: Reduced Mn valence at the La0.9Sr0.1MnO3/SrTiO3interface. (a) The background-subtracted and gain-corrected Mn-L2,3edge spectra averaged parallel to the interface. (b) Two distinct components are extracted by multivariate curve resolution. For the interface component, the major peaks of the Mn L-edge are shifted to lower energies, indicative of a reduced Mn valence. The Mn spectra across the spectroscopic image are fit to the two components as shown binned in (c) and in the full 2-D map in (d). (e) Concentration map plotting Ti, Mn and La in blue, green and red, respectively. Scale bar, 1 nm. Figure 2: Reduced Mn valence at the La 0.9 Sr 0.1 MnO 3 /SrTiO 3 interface. ( a ) The background-subtracted and gain-corrected Mn-L 2,3 edge spectra averaged parallel to the interface. ( b ) Two distinct components are extracted by multivariate curve resolution. For the interface component, the major peaks of the Mn L-edge are shifted to lower energies, indicative of a reduced Mn valence. The Mn spectra across the spectroscopic image are fit to the two components as shown binned in ( c ) and in the full 2-D map in ( d ). ( e ) Concentration map plotting Ti, Mn and La in blue, green and red, respectively. Scale bar, 1 nm. Full size image Charge quantification across the metal–insulator transition To probe how the charge transfer varies across the metal–insulator transition, this analysis was extended to the full series of LSMO films from x =0 to x =0.5. The 2-D concentration maps shown in Fig. 3a indicate that the considerable A -site intermixing at the LaMnO 3 /SrTiO 3 interface did not persist for the strontium-doped films. To characterize the manganese valence at the interface, we performed a non-negative non-linear least squares fit of the manganese signal across the interface to reference spectra for Mn +3 , Mn +3.5 and Mn +2 , Fig. 3b , obtained from the bulk LaMnO 3 , La 0.5 Sr 0.5 MnO 3 films and the literature [35] , respectively. We note that while the Mn +3.5 spectrum represents a superposition of Mn +3 and Mn +4 spectra, the mathematical decomposition of the full data set into this spectral basis is equivalent to that which could be achieved using a basis including the Mn +4 spectrum. The residuals from the fits are presented in Supplementary Fig. 9 , demonstrating the reliability of the fits across the series of samples with the basis spectra chosen. A statistically significant concentration of Mn +2 is observed at the interface for x <0.3. Furthermore, the line profiles, Fig. 3c , show a significant change in manganese valence near the interface, even in the absence of the Mn +2 component for the x= 0.3 interface. 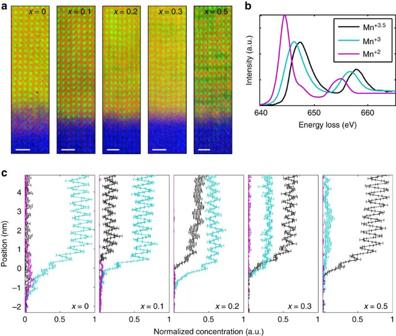Figure 3: Mn valence changes at the series of La1−xSrxMnO3/SrTiO3interfaces. Spectroscopic images forx=0, 0.1, 0.2, 0.3 and 0.5 films are shown left to right in (a). Ti is plotted in blue, Mn in green and La in red. Thex=0.5 image shows cation ordering not observed in the other films. (b) Three Mn reference spectra for Mn+2, Mn+3and Mn+3.5, used to determine the Mn valence across the interface. (c) The results of the non-negative non-linear least squares fit of the components in (b) forx=0, 0.1, 0.2, 0.3 and 0.5 ordered left to right. Error bars plot the s.e. of the mean generated from five binned regions from each spectroscopic image. Scale bar, 1 nm. Figure 3: Mn valence changes at the series of La 1− x Sr x MnO 3 /SrTiO 3 interfaces. Spectroscopic images for x =0, 0.1, 0.2, 0.3 and 0.5 films are shown left to right in ( a ). Ti is plotted in blue, Mn in green and La in red. The x =0.5 image shows cation ordering not observed in the other films. ( b ) Three Mn reference spectra for Mn +2 , Mn +3 and Mn +3.5 , used to determine the Mn valence across the interface. ( c ) The results of the non-negative non-linear least squares fit of the components in ( b ) for x= 0, 0.1, 0.2, 0.3 and 0.5 ordered left to right. Error bars plot the s.e. of the mean generated from five binned regions from each spectroscopic image. Scale bar, 1 nm. Full size image The total electronic charge transfer to the manganese ions near the interface can be calculated by subtracting the measured valence from the nominal bulk. 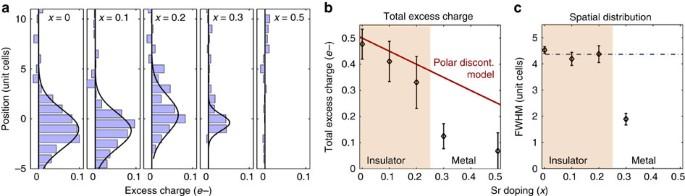Figure 4: Excess charge accumulation at the manganite–titanate interfaces. The excess charge can be computed from the deviation between the nominal bulk and the measured Mn valence across the interface. (a) The total excess charge per unit cell is plotted across the interface forx=0, 0.1, 0.2, 0.3 and 0.5 ordered left to right. The ‘0’ position denotes the interface, defined by the midpoint of the Mn concentration profile. A Gaussian fit was added as a guide to the eye. (b) The total excess charge integrated across the interface and compared with the polar discontinuity model. For insulating manganite films, the total charge observed quantitatively agrees with that needed to cancel the polar catastrophe. As the manganite becomes metallic forx≥0.3, the total charge build-up drops substantially. (c) The full width at half maximum of the Gaussian charge profiles fromashows a discontinous drop at the insulator-metal transition. A dashed line is added through the mean width for the insulating samples at 4.4 unit cells. Error bars are the s.e. of the mean. Figure 4a shows the computed charge transfer across the interface, which is integrated to find the total charge transfer in Fig. 4b . We demonstrate a quantitative agreement between the polar catastrophe electronic reconstruction model in Supplementary Fig. 2 and the measured charge on the interfacial manganese sites for x ≤0.2. For x ≥0.3, significantly less charge is measured with no statistically significant electronic transfer for x =0.5 despite the prediction of 0.25 e− . We note that this sharp discontinuity as a function of doping in the measured charge build-up at the interface coincides with the room temperature metal–insulator transition at x= 0.3. In metallic films, electronic charge transfer to the interface is expected to equilibrate the chemical potentials and to balance interface charges. The magnitude of the interface charge can be different from the polar catastrophe model because the simple ionic picture is no longer valid to describe the electrostatic potential. It is, therefore, not surprising that the magnitude of the compensating charge required for the metallic films deviates from that expected for insulating films. Figure 4: Excess charge accumulation at the manganite–titanate interfaces. The excess charge can be computed from the deviation between the nominal bulk and the measured Mn valence across the interface. ( a ) The total excess charge per unit cell is plotted across the interface for x =0, 0.1, 0.2, 0.3 and 0.5 ordered left to right. The ‘0’ position denotes the interface, defined by the midpoint of the Mn concentration profile. A Gaussian fit was added as a guide to the eye. ( b ) The total excess charge integrated across the interface and compared with the polar discontinuity model. For insulating manganite films, the total charge observed quantitatively agrees with that needed to cancel the polar catastrophe. As the manganite becomes metallic for x ≥0.3, the total charge build-up drops substantially. ( c ) The full width at half maximum of the Gaussian charge profiles from a shows a discontinous drop at the insulator-metal transition. A dashed line is added through the mean width for the insulating samples at 4.4 unit cells. Error bars are the s.e. of the mean. Full size image Charge delocalization across the metal–insulator transition Finally, we note that not only does the total electronic charge transfer to the interface change in the proximity of the metal–insulator transition, but also the width of the reconstructed region. As shown in Fig. 4c , despite the decrease in transferred charge with increasing x , the width of the electronic reconstruction region remains roughly constant for x ≤0.2 with the width of the charge profiles constant at 4.4 unit cells. Surprisingly, the significant intermixing observed for the LaMnO 3 /SrTiO 3 interface in comparison to the other films did not impact the width of charge transfer. In contrast, the small amount of charge transferred to the x =0.3 interface has a narrower width with modulations observed only over two unit cells. This length scale in the metallic state is consistent with previous theoretical [36] and experimental [37] measurements of screening lengths of ~1-2 unit cells for x =−0.33 LSMO films. Thus, both the magnitude and the spatial width of the excess electrons at the LSMO/STO interface are tuned across this phase transition. In summary, we probed a series of La 1− x Sr x MnO 3 thin films on SrTiO 3 ranging from the paramagnetic insulating to ferromagnetic metallic regions of the phase diagram. By mapping the valence changes of the manganese sites across the interface, we show a quantitative agreement between the total electron transfer to the interface for the insulating region of the phase diagram and a significantly reduced charge transfer for the metallic films. Moreover, we measured the spatial extent of the resultant excess electrons residing at the interface. Despite differences in chemical intermixing, the electronic reconstruction width remains constant at about four unit cells for the insulating films, yet narrows to two unit cells as LSMO becomes metallic. The engineering of the spatial extent of the interface charge should be useful in the construction of novel electronic phases at oxide interfaces. Thin film fabrication We investigate thin films of La 1− x Sr x MnO 3 with x =0, 0.1, 0.2, 0.3 and 0.5 grown by pulsed laser deposition on TiO 2 -terminated 0.01 wt% Nb-doped SrTiO 3 {100} substrates. For each structure, the substrate was pre-annealed under 5 × 10 −6 Torr of oxygen partial pressure ( P O 2 ) at 950 °C for 30 min after which the La 1− x Sr x MnO 3 (LSMO) thin film was deposited at a laser fluence of 0.4 J cm −2 using a KrF excimer laser at a growth temperature of 750 °C and P O 2 of 1 × 10 −3 Torr. Electron microscopy and spectroscopy Cross-sectional TEM specimens were investigated on the 5 th -order aberration corrected 100 keV Nion UltraSTEM equipped with an Enfina spectrometer. The microscope conditions were optimized for EELS spectroscopic imaging with a probe size of ~1 Å, EELS energy resolution of ~0.6 eV and a dispersion of 0.3 eV per channel. Elemental concentrations and bonding information were extracted from the simultaneous acquisition of the Ti-L 2,3 , Mn-L 2,3 , O-K and La-M 4,5 edges. To measure the concentration of all the cations in the system, the Nion UltraSTEM, now equipped with a Quefina Dual-EELS spectrometer, was used to measure the Sr-L 2,3 edge simultaneously with the Ti, Mn and La edges. For all samples, the Ti signal from the substrate and the La edges were used to accurately calibrate the energy shift and dispersion between the samples. Further details of the data acquisition and processing is given in Supplementary Discussion and the corresponding Supplementary Fig. 10 . How to cite this article: Mundy, J. A. et al. Visualizing the interfacial evolution from charge compensation to metallic screening across the manganite metal–insulator transition. Nat. Commun. 5:3464 doi: 10.1038/ncomms4464 (2014).